Complement anaphylatoxin C3a is a potent inducer of embryonic chick retina regeneration Identifying the initiation signals for tissue regeneration in vertebrates is one of the major challenges in regenerative biology. Much of the research thus far has indicated that certain growth factors have key roles. Here we show that complement fragment C3a is sufficient to induce complete regeneration of the embryonic chick retina from stem/progenitor cells present in the eye, independent of fibroblast growth factor receptor signaling. Instead, C3a induces retina regeneration via STAT3 activation, which in turn activates the injury- and inflammation-responsive factors, IL-6, IL-8 and TNF-α. This activation sets forth regulation of Wnt2b , Six3 and Sox2 , genes associated with retina stem and progenitor cells. Thus, our results establish a mechanism for retina regeneration based on injury and inflammation signals. Furthermore, our results indicate a unique function for complement anaphylatoxins that implicate these molecules in the induction and complete regeneration of the retina, opening new avenues of experimentation in the field. Components of the complement system play a major role in innate immunity and inflammation, but in recent years they have also received much attention because of their multifaceted functions in processes outside of the immune system, including the regulation of neurogenesis [1] , stem cell homing and migration [2] , [3] , [4] , [5] synapse remodelling [6] , neural crest migration [7] , cell proliferation, survival [8] , [9] and liver regeneration [10] , [11] , [12] , [13] , [14] . There is also emerging evidence that the complement system has a role in development and/or protection of the nervous system [15] , [16] . For example, the complement system may decrease inflammation in the brain instead of promoting it by reducing the production of inflammatory cytokines and increasing production of microglial neuronal growth factor [16] . In addition, astroglia, oligodendrocytes and neurons produce complement components including their receptors de novo [17] , further supporting a role for complement other than promoting inflammation. Complement component 3 (C3) and Complement component 5 (C5) are two major factors that have been investigated for their role outside of the immune system [18] . C3 is a common downstream component of all canonical complement activation mechanisms, and its cleavage into C3a and C3b is necessary for activation of C5. Mice deficient in C3 or C5 have impaired liver regeneration [11] following partial hepatectomy. Further investigation revealed C3a and the active cleavage product of C5, C5a, are necessary for the initial proliferation of hepatocytes [11] . C3a has also shown to be important for the clearance of injured tissues [12] . Moreover, expression of C3 mRNA and presence of the protein have been detected in the regenerating limb blastema and regenerating lens vesicles of urodele amphibians [19] , [20] , suggesting a more general role for C3 in regeneration. We have a powerful system for studying neuronal regeneration using the embryonic chick eye. The chick has the ability to regenerate a complete retina if the original retina is removed at embryonic day (E) 4 to 4.5. An undifferentiated neuroepithelium (NE) forms in just 3 days and a laminated retina complete with all retinal neurons and Müller glia is formed in 7 days post retinectomy (PR). Retina regeneration can occur through activation of stem/progenitor cells housed in the anterior ciliary margin (CM) of the eye or through transdifferentiation of the retinal pigmented epithelium (RPE). Activation of the CM stem/progenitor cells and the transdifferentiation of the RPE occur simultaneously, however, the regenerated retina from each mode can be distinguished allowing us to systematically study the induction of each mechanism [21] . For this study, we focused on retina regeneration arising from the stem/progenitor cells of the CM. Even though retina regeneration is possible in the embryonic chick, it does not occur spontaneously, but must be induced by the addition of exogenous factors [21] , [22] , [23] , [24] . The embryonic chick eye provides a unique model to test factors and drugs for their potential to induce neural regeneration, and to dissect the molecular mechanisms involved in the process. Information obtained could then be used for further testing in other vertebrate models including mammals. As retina regeneration in the embryonic chick occurs via two different cell sources simultaneously and is also restricted to embryonic stages, the system is limited to the study of early inductive events of regeneration, and not to test functional retina regeneration. To date, fibroblast growth factor 2 (FGF2) has been the key inducer of retina regeneration in the chick [21] , [22] , [23] , [25] , [26] . Other growth factors such as Sonic hedgehog and bone morphogenetic protein can also induce retina regeneration from the CM but a basal level of FGF2 is also required [24] , [25] . However, in this study we show that upon retina removal and addition of C3a, the retina regenerates from the activation of retinal stem and progenitor cells. We further show a new mechanism of inducing retina regeneration that does not require FGF2 signaling. This new mode of induction shows that C3a signals through its G-coupled receptor, C3aR, to stimulate retina regeneration by initially increasing the inflammatory cytokine, IL-6, through MAPK-STAT3 activation, leading to the eventual regulated expression of retinal stem and progenitor genes conducive to retina regeneration. Complement components are expressed in chick embryos Chick eyes at E4 (stage at which retinectomies are performed) express complement components C3 , Factor D and Factor B , which are required for the assembly of the alternative pathway C3 convertase (C3bBb) that cleaves C3 into C3a and C3b ( Supplementary Fig. S1a,b ). In addition, western analysis of eye tissues, using an antibody specific for the alpha-chain of chicken C3, show the presence of the 68-kDa iC3b fragment indicating C3 activation in the eyes ( Supplementary Fig. S1c ). Even though C3a is simultaneously generated during C3 activation, it is difficult to be detected by western blotting because of its low abundance, which is common to most physiological conditions [27] . In addition to C3 activation products, C3a receptor (C3aR) mRNA and protein are present in E4 eye tissues ( Supplementary Fig. S1a–c ). Immunohistochemistry confirmed the presence of C3 and C3aR in E4 eyes ( Supplementary Fig. S1d ). Interestingly, C3 mRNA is not expressed in intact CM, RPE or NE, however, C3 is observed at the protein level in all three tissues indicating the C3 produced by other cell types in the eye (mRNA in whole eye; Supplementary Fig. S1b ), or present in the egg ( Supplementary Fig. S1c ), may diffuse and bind to cells in these tissues. Furthermore, in response to injury (retinectomy), C3 mRNA is produced de novo in the CM (tissue responsible for retina regeneration; Supplementary Fig. S2a ). This increase in mRNA was not translated into a detectable increase in activated C3 in E4 eyes ( Supplementary Fig. S2b,c ). The presence of C3/C3aR proteins in the chick eye suggests that these complement components may be important in the regulation of retina development and regeneration. C3a and C3a-p induce retina regeneration To test the hypothesis that C3a has a role during retina regeneration, we performed retinectomies at E4 and then added to the eye cup, either recombinant chicken C3a, or a 21-amino-acid peptide corresponding to the carboxy terminal region of chicken C3a (C3a-p). C3a-p was used due to its ability to bind and activate the C3aR in various species [28] ( Supplementary Fig. S3 ). The embryos were collected at 3 days PR and analysed histologically for regeneration. Surprisingly, we found that both C3a and C3a-p, were sufficient to induce retina regeneration from stem/progenitor cells located in the CM in the absence of any other exogenous growth factors ( Fig. 1a,b ). FGF2 was used as a standard control throughout this study ( Fig. 1c ). A peptide of scrambled C3a-p sequence (Scr), used as a negative control, was unable to induce regeneration ( Fig. 1d ). Furthermore, C5a, a component downstream of C3a in the complement cascade was also able to induce regeneration in the absence of exogenous growth factors, further supporting a role for the complement system in retina regeneration ( Supplementary Fig. S4 ). 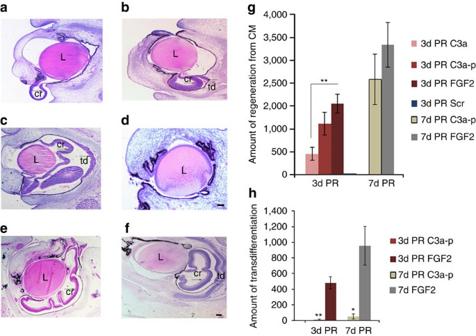Figure 1: C3a induces chick retina regeneration. (a–d) Histological analysis at 3 days (d) PR after treatment with either C3a (a), the carboxy terminus of C3a (C3a-p) (b), FGF2 (c) or a scrambled C3a fragment (Scr) (d). (e,f) Histological analysis at 7d PR after treatment with C3a-p (e) or FGF2 (f). Scale bar, 100 μm (a–f). Scale bar infalso applies toa–cande. (g) Statistical analysis of the quantification of regeneration from the CM comparing C3a (n=7 with 5/7 showing regeneration); C3a-p (n=11 at 3d PR with 9 showing regeneration andn=12 at 7d PR with 8 showing regeneration) and FGF2 treatment (n=10 at 3d PR with 10 showing regeneration andn=10 at 7d PR with 9 showing regeneration). The regeneration induced by the entire C3a fragment was significantly lower than that induced by FGF2 at 3d PR (P=0.0045) using a two-tailed permutation test. Error bars represent s.e.m. (h) Statistical analysis of the quantification of regeneration comparing the regeneration from transdifferentation of the RPE in response to C3a-p and FGF2. Transdifferentiation in C3a-p-treated eyes was significantly less than that in FGF2-treated eyes at both 3d (P=0.0012) and 7d PR (P=0.0182) using a two-tailed permutation test. *P<0.05 and **P<0.01. The mean amount of regeneration from the CM and transdifferentiation as well as the s.e.m. and range are provided inSupplementary Table S7. cr, regeneration from the CM; td, RPE transdifferentiation; L, lens. Figure 1: C3a induces chick retina regeneration. ( a – d ) Histological analysis at 3 days (d) PR after treatment with either C3a ( a ), the carboxy terminus of C3a (C3a-p) ( b ), FGF2 ( c ) or a scrambled C3a fragment (Scr) ( d ). ( e , f ) Histological analysis at 7d PR after treatment with C3a-p ( e ) or FGF2 ( f ). Scale bar, 100 μm ( a – f ). Scale bar in f also applies to a – c and e . ( g ) Statistical analysis of the quantification of regeneration from the CM comparing C3a ( n =7 with 5/7 showing regeneration); C3a-p ( n =11 at 3d PR with 9 showing regeneration and n =12 at 7d PR with 8 showing regeneration) and FGF2 treatment ( n =10 at 3d PR with 10 showing regeneration and n =10 at 7d PR with 9 showing regeneration). The regeneration induced by the entire C3a fragment was significantly lower than that induced by FGF2 at 3d PR ( P =0.0045) using a two-tailed permutation test. Error bars represent s.e.m. ( h ) Statistical analysis of the quantification of regeneration comparing the regeneration from transdifferentation of the RPE in response to C3a-p and FGF2. Transdifferentiation in C3a-p-treated eyes was significantly less than that in FGF2-treated eyes at both 3d ( P =0.0012) and 7d PR ( P =0.0182) using a two-tailed permutation test. * P <0.05 and ** P <0.01. The mean amount of regeneration from the CM and transdifferentiation as well as the s.e.m. and range are provided in Supplementary Table S7 . cr, regeneration from the CM; td, RPE transdifferentiation; L, lens. Full size image Even though there was no significant difference in the level of regeneration between C3a and C3a-p, C3a did induce significantly less regeneration than FGF2 (our standard procedure used for comparison [21] , [25] ; Fig. 1a–c,g ). Given that the full-length C3a is a recombinant protein, it is likely that insufficient protein refolding may affect C3a activity. For this reason, we chose to use C3a-p in all subsequent experiments. The amount of regeneration from the CM induced by C3a-p at 3 and 7 days PR was comparable to the regeneration induced by FGF2 ( Fig. 1b,c,e–g ). While both transdifferentiation of the RPE and regeneration from stem/progenitor cells of the CM occurred in response to C3a-p, our data showed that regeneration from the CM was much more robust ( Fig. 1g,h ). Thus, we chose to further examine in detail the role of C3a-p in the activation of cells from the CM. At the cellular level, the mature retina is organized in three main layers: the ganglion cell layer; the inner nuclear layer with amacrine, bipolar and horizontal cells; and the outer nuclear layer containing photoreceptors. In addition, Müller glia cells expand throughout the three cell layers. Interestingly, C3a-p treatment generated all the cell types of the retina, including Müller glia in retinectomized eyes ( Fig. 2a ). In fact, C3a-p actually generated a significantly higher number of bipolar and amacrine cells when compared with the number generated by FGF2 treatment and with the number present in an equivalent retina at embryonic day 11 (E11; Fig. 2b ). Notably, C3aR is co-expressed with AP-2 in amacrine cells suggesting one possible reason why a higher number of amacrine cells is observed. However, C3aR is not co-expressed with Chx-10 in bipolar cells indicating that the expression of C3aR may not be directly necessary for the increased differentiation of this cell type ( Fig. 2c ). Injection of BrdU into C3a-p-treated regenerating eyes 1 h before collection, indicated that the number of cells in S phase are significantly increased in the posterior region of the regenerating retina at 3 and 7 days PR when compared with the number induced by FGF2 ( Fig. 3a,b ). In addition, we discovered an increase in the number of progenitor cells (identified by co-expression of Pax-6 and Chx-10) in the regenerating retinas induced by C3a-p when compared with those induced by FGF2 ( Fig. 3c,d ). This increase in the number of progenitors, most likely contributes to the increase in the number of proliferating cells and provides an alternative explanation for the increase in the number of differentiated amacrine and bipolar cells seen in C3a-p-induced retinas. These particular cells may have been selectively increased due to the fact that progenitors were produced and ready to differentiate at the correct developmental time for their differentiation [29] ( Fig. 2b ). 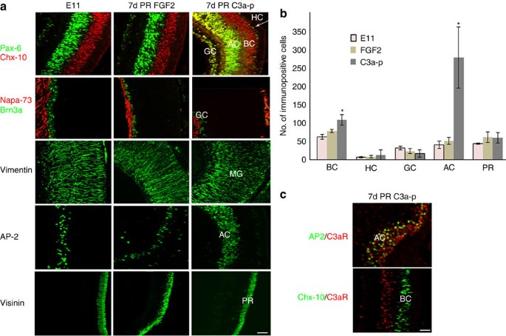Figure 2: C3a-p regenerates a retina from the CM with all retinal cell types present. (a) Immunohistochemical staining using antibodies against cell-specific markers at 7 days (d) PR. Retinal cell types in a developmentally equivalent eye (E11) as well as retinal cell types regenerated in response to FGF2 are shown for comparison. Pax-6 (green) is a specific marker for ganglion (GC), amacrine (AC) and horizontal cells (HC); Chx-10 (red) is a specific marker for bipolar cells (BC). Napa-73 (red) is specific for ganglion cell axons and Brn-3a (green) is specific for GC. Vimentin is specific for Müller glia (MG) cells, AP-2 is specific for AC and visinin is specific for photoreceptors (PR). Images are sections from the posterior region of the eye (seeSupplementary Fig. S1afor eye schematic). The scale bar in the last panel represents 20 μm and applies to all panels. (b) Statistical analysis of the number of each retinal cell type shows that there is a significant increase in AC (P=0.01) and BC (P=0.03) in the regenerated retina in C3a-p-treated eyes when compared with the FGF2-treated eyes. The number of GC was determined by counting Brn3a+cells; the number of AC was determined by counting the number of AP-2+cells; the number of BC by Chx-10 staining; HC by Pax-6 and PR by visinin staining (n=5 different eyes). A two-tailed permutation test was used for statistical analysis. Error bars represent s.e.m. The mean number of immunopositive cells, s.e.m. and range are given inSupplementary Table S8. *P<0.05. (c) Immunohistochemistry shows that AP-2 (green) and the C3aR (red) are co-expressed in some AC in C3a-p-treated eyes 7d PR, while Chx-10 marking BC and C3aR are not. The scale bar in the last panel represents 20 μm and applies to both panels. Figure 2: C3a-p regenerates a retina from the CM with all retinal cell types present. ( a ) Immunohistochemical staining using antibodies against cell-specific markers at 7 days (d) PR. Retinal cell types in a developmentally equivalent eye (E11) as well as retinal cell types regenerated in response to FGF2 are shown for comparison. Pax-6 (green) is a specific marker for ganglion (GC), amacrine (AC) and horizontal cells (HC); Chx-10 (red) is a specific marker for bipolar cells (BC). Napa-73 (red) is specific for ganglion cell axons and Brn-3a (green) is specific for GC. Vimentin is specific for Müller glia (MG) cells, AP-2 is specific for AC and visinin is specific for photoreceptors (PR). Images are sections from the posterior region of the eye (see Supplementary Fig. S1a for eye schematic). The scale bar in the last panel represents 20 μm and applies to all panels. ( b ) Statistical analysis of the number of each retinal cell type shows that there is a significant increase in AC ( P =0.01) and BC ( P =0.03) in the regenerated retina in C3a-p-treated eyes when compared with the FGF2-treated eyes. The number of GC was determined by counting Brn3a + cells; the number of AC was determined by counting the number of AP-2 + cells; the number of BC by Chx-10 staining; HC by Pax-6 and PR by visinin staining ( n =5 different eyes). A two-tailed permutation test was used for statistical analysis. Error bars represent s.e.m. The mean number of immunopositive cells, s.e.m. and range are given in Supplementary Table S8 . * P <0.05. ( c ) Immunohistochemistry shows that AP-2 (green) and the C3aR (red) are co-expressed in some AC in C3a-p-treated eyes 7d PR, while Chx-10 marking BC and C3aR are not. The scale bar in the last panel represents 20 μm and applies to both panels. 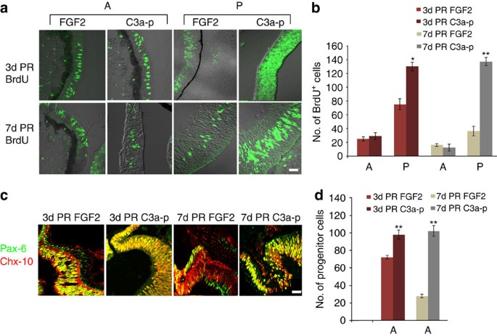Figure 3: C3a induces proliferation and increases the number of retinal progenitors during chick retina regeneration. (a) BrdU incorporation shown in the anterior (A) and posterior (P) regions of the regenerating retina from the CM 3 and 7 days (d) PR, and after induction with C3a-p. (Please refer to the eye schematic inSupplementary Fig. S1afor localization of the anterior and posterior regions). The RPE and PE sometimes dissociate from the regenerating retina and from the CM, and for this reason, they are not visible in all images. The scale bar in the last panel represents 20 μm and applies to all panels. BrdU incorporation in the regenerating retina after treatment with FGF2 is shown for comparison. (b) Quantitative analysis of the number of BrdU+cells shows that there are significantly more BrdU+cells in the posterior region of the regenerating retina in C3a-p-treated eyes than in FGF2-treated eyes (P=0.03 at 3d PR andP=0.007 at 7d PR;n=5 different eyes). A two-tailed permutation test was used for statistical analysis. Error bars represent s.e.m. The mean number of BrdU+cells for each treatment is given inSupplementary Table S8. (c) Immunohistochemical staining using antibodies against Pax-6 (green) and Chx-10 (red) shows the number of retinal progenitor cells present in the anterior region (A) of eyes treated with C3a-p at 3 and 7d PR. Co-expression of both Pax-6/Chx-10 is indicative of retinal progenitor cells (yellow). The number of progenitors in FGF2-treated eyes is shown for comparison. The scale bar in the last panel represents 20 μm and applies to all panels. (d) Quantitative analysis of (c) shows that there is a significant increase in the number of progenitors in the anterior region of the regenerated retina in eyes treated with C3a-p when compared with eyes treated with FGF2 at both time points (P=0.008 at 3d PR andP=0.006 at 7d PR;n=5 different eyes). A two-tailed permutation test was used for statistical analysis. Error bars represent s.e.m. The mean number of Chx-10/Pax-6 immunopositive cells along, with s.e.m. and range is given inSupplementary Table S8. *P<0.05; **P<0.01. Full size image Figure 3: C3a induces proliferation and increases the number of retinal progenitors during chick retina regeneration. ( a ) BrdU incorporation shown in the anterior (A) and posterior (P) regions of the regenerating retina from the CM 3 and 7 days (d) PR, and after induction with C3a-p. (Please refer to the eye schematic in Supplementary Fig. S1a for localization of the anterior and posterior regions). The RPE and PE sometimes dissociate from the regenerating retina and from the CM, and for this reason, they are not visible in all images. The scale bar in the last panel represents 20 μm and applies to all panels. BrdU incorporation in the regenerating retina after treatment with FGF2 is shown for comparison. ( b ) Quantitative analysis of the number of BrdU + cells shows that there are significantly more BrdU + cells in the posterior region of the regenerating retina in C3a-p-treated eyes than in FGF2-treated eyes ( P =0.03 at 3d PR and P =0.007 at 7d PR; n =5 different eyes). A two-tailed permutation test was used for statistical analysis. Error bars represent s.e.m. The mean number of BrdU + cells for each treatment is given in Supplementary Table S8 . ( c ) Immunohistochemical staining using antibodies against Pax-6 (green) and Chx-10 (red) shows the number of retinal progenitor cells present in the anterior region (A) of eyes treated with C3a-p at 3 and 7d PR. Co-expression of both Pax-6/Chx-10 is indicative of retinal progenitor cells (yellow). The number of progenitors in FGF2-treated eyes is shown for comparison. The scale bar in the last panel represents 20 μm and applies to all panels. ( d ) Quantitative analysis of ( c ) shows that there is a significant increase in the number of progenitors in the anterior region of the regenerated retina in eyes treated with C3a-p when compared with eyes treated with FGF2 at both time points ( P =0.008 at 3d PR and P =0.006 at 7d PR; n =5 different eyes). A two-tailed permutation test was used for statistical analysis. Error bars represent s.e.m. The mean number of Chx-10/Pax-6 immunopositive cells along, with s.e.m. and range is given in Supplementary Table S8 . * P <0.05; ** P <0.01. Full size image C3a-p induces regeneration independent of FGF signaling FGF2 is considered a critical molecule for the induction of retina regeneration in the chick. However, data from RT–qPCR at 2 h PR indicated that C3a-p does not stimulate the expression of FGF2 in the CM above the level induced by retinectomy alone, which is not sufficient to induce regeneration ( Fig. 4a ). Likewise, FGF2 does not increase the expression of C3 or C3aR at 2 h PR further demonstrating that C3a-p and FGF2 have independent modes to trigger regeneration ( Supplementary Fig. S5 ). However, FGF2 expression was significantly stimulated by C3a-p 24 h later, suggesting that the FGF pathway most likely has a role in events post induction including proliferation, differentiation and cell survival [25] ( Fig. 4a ). 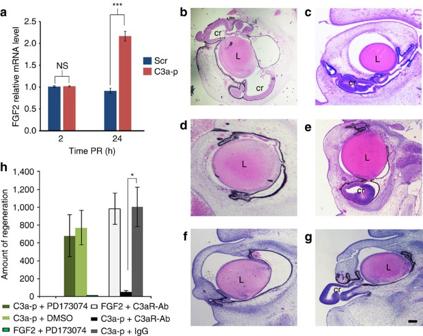Figure 4: C3a-p induction of chick retina regeneration is independent of FGF2. (a) RT–qPCR shows the level ofFGF2expression stimulated by treatment with C3a-p in the CM at 2 h PR and 24 h PR. The level ofFGF2expression was normalized to the level expressed in the CM of eyes undergoing retinectomy without treatment. Error bars represent s.e.m. The mean ratio ofFGF2expression toGAPDHexpression, together with the s.e.m. and range, is provided inSupplementary Table S5. Significance was determined by comparing the expression ofFGF2in eyes treated with C3a-p to that in eyes treated with scrambled peptide (Scr).P-value=0.0003 using the Student’st-test.;n=3 biological samples done in triplicate. ***P<0.001. (b–g) Histological analysis at 3 days (d) PR after treatment with C3a-p+PD173074 (b), C3a-p+DMSO (c), FGF2+PD173074 (d). FGF2+an antibody that blocks the C3a receptor (C3aR-Ab) (e), C3a-p+C3aR-Ab (f), or C3a-p+pre-immune serum for C3aR (IgG) (g). The scale bar in (g) represents 100 μm and also applies to (b–f). (h) Quantification of regeneration shows there is a significant difference in the amount of regeneration between eyes treated with C3a-p+IgG (n=7; 5 with regeneration) and C3a-p+C3aR-Ab (n=9; 1 with regeneration) (P-value=0.0376 using a two-tailed permutation test). There is also significant difference in the amount of regeneration between eyes treated with FGF2 and those treated with FGF2+PD173074 (n=5; 0 with regeneration) (P=0.0011 using a two-tailed permutation test). *P<0.05. Error bars represent s.e.m.n=9; 7 with regeneration for C3a-p+DMSO-treated eyes,n=8; 6 with regeneration for C3a-p+PD173074-treated eyes andn=14; 12 with regeneration for FGF2+C3aR-Ab-treated eyes. The mean amount of regeneration, s.e.m. and range are provided inSupplementary Table S7. NS, not significant; cr, regeneration from the ciliary margin; L, lens. Figure 4: C3a-p induction of chick retina regeneration is independent of FGF2. ( a ) RT–qPCR shows the level of FGF2 expression stimulated by treatment with C3a-p in the CM at 2 h PR and 24 h PR. The level of FGF2 expression was normalized to the level expressed in the CM of eyes undergoing retinectomy without treatment. Error bars represent s.e.m. The mean ratio of FGF2 expression to GAPDH expression, together with the s.e.m. and range, is provided in Supplementary Table S5 . Significance was determined by comparing the expression of FGF2 in eyes treated with C3a-p to that in eyes treated with scrambled peptide (Scr). P- value=0.0003 using the Student’s t -test. ; n =3 biological samples done in triplicate. *** P <0.001. ( b – g ) Histological analysis at 3 days (d) PR after treatment with C3a-p+PD173074 ( b ), C3a-p+DMSO ( c ), FGF2+PD173074 ( d ). FGF2+an antibody that blocks the C3a receptor (C3aR-Ab) ( e ), C3a-p+C3aR-Ab ( f ), or C3a-p+pre-immune serum for C3aR (IgG) ( g ). The scale bar in ( g ) represents 100 μm and also applies to ( b – f ). ( h ) Quantification of regeneration shows there is a significant difference in the amount of regeneration between eyes treated with C3a-p+IgG ( n =7; 5 with regeneration) and C3a-p+C3aR-Ab ( n =9; 1 with regeneration) ( P -value=0.0376 using a two-tailed permutation test). There is also significant difference in the amount of regeneration between eyes treated with FGF2 and those treated with FGF2+PD173074 ( n =5; 0 with regeneration) ( P =0.0011 using a two-tailed permutation test). * P <0.05. Error bars represent s.e.m. n =9; 7 with regeneration for C3a-p+DMSO-treated eyes, n =8; 6 with regeneration for C3a-p+PD173074-treated eyes and n =14; 12 with regeneration for FGF2+C3aR-Ab-treated eyes. The mean amount of regeneration, s.e.m. and range are provided in Supplementary Table S7 . NS, not significant; cr, regeneration from the ciliary margin; L, lens. Full size image To further support the hypothesis that C3a-p-induced regeneration is initially independent of FGF2, we performed retinectomies at E4 and then added C3a-p along with an inhibitor for FGF receptors (PD173074). Inhibiting FGF receptor (FGFR) activity did not affect the regeneration induced by C3a-p. Equivalent regeneration was seen at 3 days PR in the presence or absence of the inhibitor ( Fig. 4b,c,h ). PD173074 was able to inhibit FGF2-induced regeneration ( Fig. 4d,h ), demonstrating the specificity of the inhibitor. Conversely, inhibition of the C3aR by the addition of a C3a receptor-specific antibody (C3aR-Ab) had no significant effect on the induction of regeneration by FGF2, but it did inhibit regeneration induced by C3a-p ( Fig. 4e,f,h ). The presence of pre-immune serum (IgG) during C3a-p-induced regeneration had no effect ( Fig. 4g,h ). These results indicate that C3a-p is using a novel and hitherto unsuspected mechanism to induce retina regeneration, independent of the FGFR pathway. C3a-p induces regeneration via C3aR-MAPK-STAT3 signaling This possibility prompted us to look for an alternative mechanism of induction. STAT3 is a multifunctional protein that, when activated, has a role in stem cell proliferation, tissue regeneration, injury and cell survival and has been shown to be a downstream target of C3a [11] , [13] , [30] , [31] . STAT3 has two phosphorylation sites: tyrosine at residue 705 (Y705) and a serine at residue 727 (ref. 32 ) (S727). Phosphorylation at serine 727 is required for the maximal transcriptional activity of STAT3 (ref. 33 ). To determine whether STAT3 is indeed activated by C3a-p during retina regeneration, we performed retinectomies at E4, added C3a-p to the eye cup, and collected protein from the CM of regenerating eyes 2 h later. For comparison, we also collected proteins from retinectomized eyes treated with Scr, as well as from eyes that received no exogenous treatment. Our initial investigation did not show an upregulation of phosphorylated Y705 STAT3, so we focused our attention on the S727 STAT3. Western blot results revealed that STAT3 phosphorylated at serine 727 (pS727 STAT3) was upregulated in eyes treated with C3a-p 2 h PR, when compared with untreated eyes or eyes treated with Scr ( Fig. 5a and Supplementary Fig. S6a ). The addition of C3aR-Ab together with C3a-p after retinectomy blocked the phosphorylation of S727 STAT3 ( Fig. 5b and Supplementary Fig. S6a ). This result indicates that the activation of STAT3 is dependent on the interaction of C3a with its receptor. 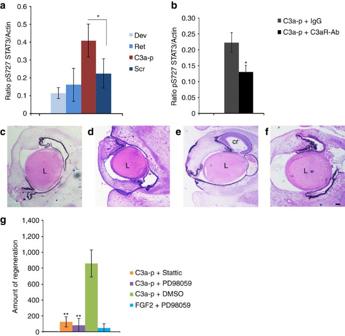Figure 5: C3a-p activates STAT3 during chick retina regeneration. (a) Western blot analysis shows the level of phosphorylation of S727 STAT3 at 2 h PR in E4 developmental eyes (Dev), retinectomized eyes with no treatment (Ret), C3a-p-treated eyes and eyes treated with Scrambled C3a (Scr).P=0.03125 using the exact binomial test comparing C3a-p treatment and Scr treatment;n=5 biological samples. (b) Western analysis shows the level of phosphorylation of S727 STAT3 (pS727 STAT3) at 2 h PR in eyes treated with C3a-p+IgG and eyes treated with C3a-p+C3aR-Ab.P=0.03125 using the exact binomial test;n=5 biological samples. Error bars represent s.e.m. The mean ratio of pS727 STAT3 to actin, s.e.m., and range are provided inSupplementary Table S3. (c–f) Histological analysis at 3 days (d) PR after treatment with either C3a-p+ Stattic (c), C3a-p+PD98059 (d), C3a-p+DMSO (e) or FGF2+PD98059 (f). (g) Quantification of the amount of regeneration at 3d PR shows that C3a-p-induced regeneration is significantly reduced in the presence of Stattic (P=0.0054;n=10) and PD98059 (P=0.0081;n=9) when compared with C3a-p+DMSO (n=9). FGF2-induced regeneration is also significantly reduced in the presence of PD98059 (n=5),P-value=0.0027 compared with FGF2-induced regeneration (Fig. 1g) *P<0.05; **P<0.01. A two-tailed permutation test was used for statistical analysis. Error bars represent s.e.m. The mean amount of regeneration, s.e.m. and range for each treatment are provided inSupplementary Table S7. cr, regeneration from the ciliary margin; L, lens. Scale bar 100 μm (c–f). Figure 5: C3a-p activates STAT3 during chick retina regeneration. ( a ) Western blot analysis shows the level of phosphorylation of S727 STAT3 at 2 h PR in E4 developmental eyes (Dev), retinectomized eyes with no treatment (Ret), C3a-p-treated eyes and eyes treated with Scrambled C3a (Scr). P =0.03125 using the exact binomial test comparing C3a-p treatment and Scr treatment; n =5 biological samples. ( b ) Western analysis shows the level of phosphorylation of S727 STAT3 (pS727 STAT3) at 2 h PR in eyes treated with C3a-p+IgG and eyes treated with C3a-p+C3aR-Ab. P =0.03125 using the exact binomial test; n =5 biological samples. Error bars represent s.e.m. The mean ratio of pS727 STAT3 to actin, s.e.m., and range are provided in Supplementary Table S3 . ( c – f ) Histological analysis at 3 days (d) PR after treatment with either C3a-p+ Stattic ( c ), C3a-p+PD98059 ( d ), C3a-p+DMSO ( e ) or FGF2+PD98059 ( f ). ( g ) Quantification of the amount of regeneration at 3d PR shows that C3a-p-induced regeneration is significantly reduced in the presence of Stattic ( P =0.0054; n =10) and PD98059 ( P =0.0081; n =9) when compared with C3a-p+DMSO ( n =9). FGF2-induced regeneration is also significantly reduced in the presence of PD98059 ( n =5), P- value=0.0027 compared with FGF2-induced regeneration ( Fig. 1g ) * P <0.05; ** P <0.01. A two-tailed permutation test was used for statistical analysis. Error bars represent s.e.m. The mean amount of regeneration, s.e.m. and range for each treatment are provided in Supplementary Table S7 . cr, regeneration from the ciliary margin; L, lens. Scale bar 100 μm ( c – f ). Full size image To confirm S727 STAT3 has a role in C3a-p-induced regeneration, we performed retinectomies and added inhibitors specific for either STAT3 or a serine/threonine kinase ( Fig. 5c–g ). Stattic, an inhibitor of the phosphorylation and dimerization of STAT3, was added along with C3a-p and tissues were collected at 3 days PR for histological analysis. We observed a significant decrease in regeneration in the presence of Stattic, supporting our western blot results ( Fig. 5c,g ). Treatment of C3a-p with DMSO resulted in regeneration equivalent to that with C3a-p alone, demonstrating that the decreased regeneration was specifically caused by the inhibitor ( Fig. 5e,g ). A serine/threonine kinase is required for STAT3 to be phosphorylated at serine 727. The serine kinase MAPK has been shown to activate STAT3 (refs 34 , 35 ), and therefore we speculated that MAPK could be activating STAT3 in our system. We performed retinectomies at E4, added C3a-p and an inhibitor of MAPK (PD98059), and collected the eyes for histological analysis at 3 days PR. C3a-p, as well as FGF2 known to induce regeneration through MAPK signaling [25] , failed to induce regeneration in the presence of PD98059, indicating that MAPK has a role in the regeneration induced by C3a-p, possibly by phosphorylating S727 STAT3 ( Fig. 5d,f,g ). Genes regulated by C3a/C3aR-MAPK-STAT3 signaling To further elucidate the molecular mechanisms involved in the induction of regeneration, we used RT–qPCR to determine which genes are regulated by pS727 STAT3. We performed retinectomies at E4, treated the eyes with C3a-p, and collected the RNA from the CM (isolated by laser-capture microdissection (LCM)) at 2 h PR. C3a has been shown to increase the expression of cytokines, as it induces inflammation in response to injury [30] , [36] . IL-6, for example, is involved in liver regeneration [11] , [13] , [30] and its gene has a binding site for STAT3 (ref. 37 ). Therefore, we investigated the regulation of IL-6 expression in C3a-p-treated eyes. RT–qPCR showed an increase in IL-6 expression at 2 h PR in the CM of eyes treated with C3a-p ( Fig. 6a ). The increase in IL-6 expression was dependent on MAPK, STAT3 and the interaction of C3a with its receptor, as treatment with PD98059, Stattic or C3aR-Ab inhibited IL-6 expression ( Fig. 6a ). The importance of IL-6 in C3a-p-induced regeneration was further analysed by histological analysis ( Fig. 6b–f ). A decrease in regeneration was seen after performing retinectomies at E4, adding C3a-p along with a specific blocking antibody against IL-6 (IL-6 Ab) [38] and assaying for regeneration at 3 days PR ( Fig. 6d–f ). The C3a-p-dependent phosphorylation of S727 STAT3 was also decreased in the presence of the IL-6 Ab, suggesting a possible feedback loop for STAT3 activation ( Fig. 6g and Supplementary Fig. S6b ). Neither the regenerative ability nor the level of pS727 STAT3 was affected by the presence of IgG ( Fig. 6e,f ). In fact, IL-6 alone was able to induce regeneration in the absence of exogenous C3a-p ( Fig. 6b,c,f ) suggesting that IL-6 acts downstream of C3a during the induction of retina regeneration. The expression of two other inflammatory factors, IL-8 and TNFα, was also significantly increased in the CM of eyes treated with C3a-p ( Supplementary Fig. S7 ). 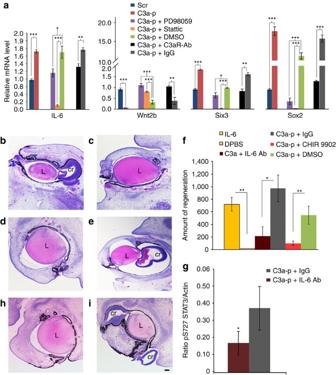Figure 6: C3a-p regulates the expression of injury-responsive genes as well as retinal stem and progenitor genes. (a)RT–qPCR shows the level of expression ofIL-6,Wnt2b,Six3andSox2in the presence of Scr, C3a-p, C3a-p+PD98059, C3a+Stattic, C3a-p+DMSO, C3a-p+C3aR-Ab or C3a-p+IgG. The expression levels were normalized to that in the CM of retinectomized eyes with no other treatment. Significance was determined by comparing C3a-p and Scr (P=0.0006, 0.000001, 0.0006, 0.0002 forIL-6, Wnt2b,Six3andSox2, respectively); C3a-p+IgG and C3a-p+C3aR-Ab (P=0.003, 0.002, 0.001, 0.0001 forIL-6,Wnt2b,Six3andSox2, respectively); C3a-p+DMSO and C3a-p+PD98059 (P=0.01, 0.0006, 0.02, 0.0001 forIL-6,Wnt2b,Six3andSox2, respectively); and C3a-p+DMSO and C3a-p+Stattic (P=0.0001, 0.0009, 0.00000006, 0.00009 forIL-6,Wnt2b,Six3andSox2, respectively);n=3 biological samples performed in triplicate. The Student’st-test was used to determine significance. Error bars represent s.e.m. The mean ratio of the mRNA for each gene of interest relative to GAPDH along with the s.e.m. and range is provided inSupplementary Table S6. *P<0.05; **P<0.01; ***P<0.001. (b–e) Histological analysis shows the amount of regeneration at 3 days (d) PR in the presence of IL-6 (b), DPBS (c), C3a-p+IL-6 Ab (d) or C3a-p+IgG (e). (f) Graphical representation of the mean level of regeneration for each histological analysis. IL-6 (n=10) versus DPBS (n=8;P=0.0020); C3a-p+IL-6 Ab (n=8) versus C3a-p+IgG (n=8;P=0.026); and C3a-p+CHIR (n=16) versus C3a-p+DMSO (n=12;P=0.0041). Statistical analysis was done using the two-tailed permutation test. Error bars represent s.e.m. *P<0.05; **P<0.01. The mean amount of regeneration, s.e.m. and range for each treatment are provided inSupplementary Table S7. (g) Western analysis shows the amount of phosphorylation of STAT3 at Ser727 (pS727 STAT3) in the presence of IL-6 Ab (P=0.03125;n=5 biological samples). *P<0.05. Statistical analysis was done using the exact binomial test. Error bars represent s.e.m. Mean ratio of pS727 STAT3 to actin, s.e.m, and range are provided inSupplementary Table S3. (h,i) Histological analysis shows the amount of regeneration in the presence of C3a-p+CHIR (h) or C3a-p+DMSO (i). cr, regeneration from the ciliary margin; L, lens. Figure 6: C3a-p regulates the expression of injury-responsive genes as well as retinal stem and progenitor genes. ( a )RT–qPCR shows the level of expression of IL-6 , Wnt2b , Six3 and Sox2 in the presence of Scr, C3a-p, C3a-p+PD98059, C3a+Stattic, C3a-p+DMSO, C3a-p+C3aR-Ab or C3a-p+IgG. The expression levels were normalized to that in the CM of retinectomized eyes with no other treatment. Significance was determined by comparing C3a-p and Scr ( P =0.0006, 0.000001, 0.0006, 0.0002 for IL-6, Wnt2b , Six3 and Sox2 , respectively); C3a-p+IgG and C3a-p+C3aR-Ab ( P =0.003, 0.002, 0.001, 0.0001 for IL-6 , Wnt2b , Six3 and Sox2 , respectively); C3a-p+DMSO and C3a-p+PD98059 ( P =0.01, 0.0006, 0.02, 0.0001 for IL-6 , Wnt2b , Six3 and Sox2 , respectively); and C3a-p+DMSO and C3a-p+Stattic ( P =0.0001, 0.0009, 0.00000006, 0.00009 for IL-6 , Wnt2b , Six3 and Sox2 , respectively); n =3 biological samples performed in triplicate. The Student’s t -test was used to determine significance. Error bars represent s.e.m. The mean ratio of the mRNA for each gene of interest relative to GAPDH along with the s.e.m. and range is provided in Supplementary Table S6 . * P <0.05; ** P <0.01; *** P <0.001. ( b – e ) Histological analysis shows the amount of regeneration at 3 days (d) PR in the presence of IL-6 ( b ), DPBS ( c ), C3a-p+IL-6 Ab ( d ) or C3a-p+IgG ( e ). ( f ) Graphical representation of the mean level of regeneration for each histological analysis. IL-6 ( n =10) versus DPBS ( n =8; P =0.0020); C3a-p+IL-6 Ab ( n =8) versus C3a-p+IgG ( n =8; P =0.026); and C3a-p+CHIR ( n =16) versus C3a-p+DMSO ( n =12; P =0.0041). Statistical analysis was done using the two-tailed permutation test. Error bars represent s.e.m. * P <0.05; ** P <0.01. The mean amount of regeneration, s.e.m. and range for each treatment are provided in Supplementary Table S7 . ( g ) Western analysis shows the amount of phosphorylation of STAT3 at Ser727 (pS727 STAT3) in the presence of IL-6 Ab ( P =0.03125; n =5 biological samples). * P <0.05. Statistical analysis was done using the exact binomial test. Error bars represent s.e.m. Mean ratio of pS727 STAT3 to actin, s.e.m, and range are provided in Supplementary Table S3 . ( h , i ) Histological analysis shows the amount of regeneration in the presence of C3a-p+CHIR ( h ) or C3a-p+DMSO ( i ). cr, regeneration from the ciliary margin; L, lens. Full size image To determine whether C3a regulates any retina-specific genes necessary for regeneration through STAT3 activation, we performed RT–qPCR at 2 and 6 h PR using RNA isolated from the CM. Interestingly, Wnt2b , a stem cell maintenance factor in the retina [39] with a binding site for STAT3 (ref. 37 ), was downregulated in the CM at 6 h PR ( Fig. 6a ). The addition of PD98059, Stattic or C3aR-Ab reversed this downregulation ( Fig. 6a ). Addition of the pharmacological agent CHIR 99021, an activator of the Wnt pathway that we show increases Wnt2b and Axin2 mRNA (two downstream targets of the Wnt pathway) in the CM after retinectomy, ( Supplementary Fig. S8 ) also reduced the ability of C3a-p to induce regeneration as shown by histological analysis at 3 days PR ( Fig. 6f,h,i ). At the same time, we saw an increase in the expression of Six3 (ref. 40 ) and Sox2 (ref. 41 ), which are retinal progenitor genes containing STAT3-binding sites [37] , [42] . This change was dependent on a functional MAPK and STAT3 pathway as well as C3aR activity, as inhibition at any of these levels resulted in a significant decrease in Six3 and Sox 2 expression ( Fig. 6a ). Together, these results demonstrate that, initially, C3a induces injury-responsive genes as expected, but then downregulates the expression of stem cell maintenance genes while inducing the expression of progenitor-specific genes, thereby setting the stage for regeneration ( Fig. 7 ). 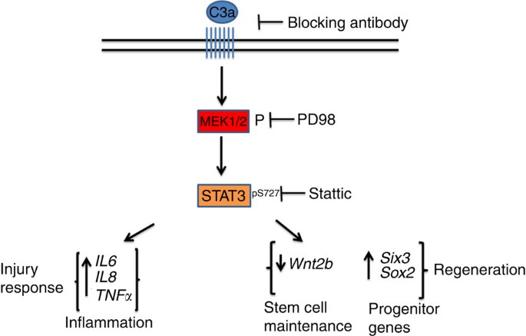Figure 7: A model for the induction of chick retina regeneration by C3a. A model depicting the mechanism of induction of retina regeneration by C3a. C3a binds its receptor, C3aR, which leads to the activation of MAPK and subsequent phosphorylation of S727 STAT3. In the presence of active pS727 STAT3, expression of injury-responsive genes,IL-6,TNF-αandIL-8is increased followed by a decrease in the expression of the retinal stem cell gene,Wnt2b, and an increase in expression of the retinal progenitor genes,Six3andSox2. Figure 7: A model for the induction of chick retina regeneration by C3a. A model depicting the mechanism of induction of retina regeneration by C3a. C3a binds its receptor, C3aR, which leads to the activation of MAPK and subsequent phosphorylation of S727 STAT3. In the presence of active pS727 STAT3, expression of injury-responsive genes, IL-6 , TNF-α and IL-8 is increased followed by a decrease in the expression of the retinal stem cell gene, Wnt2b , and an increase in expression of the retinal progenitor genes, Six3 and Sox2 . Full size image There is increasing evidence that inflammation signals are key to the initiation of regeneration [11] , [13] , [30] , [43] . In mammals, during retinal injury/disease, inflammation signals are also produced, so it would be of critical importance to understand how these signals are conducive to regeneration instead of scarring and necrosis/cell death. Mammals lack the ability to regenerate their retina, however, there are several cell types within the eye that have the potential to regenerate. These include Müller glia, cells of the RPE and CM cells. Our results in the chick eye provide insights that help explain how inflammation signals, including C3a, might direct mammalian Müller glia cells, RPE or even cells from the CM to regenerate lost retina cells. Our findings have revealed a previously unsuspected, new function of complement components that has a positive effect on eye tissue repair, in contrast to the negative effects reported during eye disease [44] . Polymorphic variants of Factor H have been linked with macular degeneration. These variants imply loss of complement Factor H activity, and thus increased complement activation [44] . We can reconcile these apparent differences by hypothesizing that the balance of complement must be tightly regulated to ensure the appropriate response. In the study presented here, we used 1 nM of C3a-p per surgery. When a higher amount of C3a-p was used, the regenerating retina was not maintained, and a significant level of apoptosis was induced by 7 days PR ( Supplementary Fig. S9 ). This suggests that there is a tight control of the pathways involved. This conclusion is supported by other studies in which complement has been reported to have negative and positive effects in the nervous system and during angiogenesis [15] , [45] , [46] . Furthermore, a regulated balance of C3a has been found to be necessary in the liver to promote regeneration instead of persistent inflammation. In fact, the dosage of C3a resulting in liver regeneration also produces an increase in IL-6 and STAT3 activation, further supporting our conclusions [30] . It is also probable that the diverse effects of complement molecules in retinal eye diseases are also ‘amount- and context-’ dependent as shown in previous studies [45] , [46] , [47] . A clear understanding of the mechanisms by which C3a induces retina repair and regeneration will help determine when and how much complement components are necessary to allow for repair versus disease. Chick embryos Specific pathogen-free (SPF) fertilized chicken eggs were purchased from Charles River Laboratories, Wilmington, MA, and incubated in a 38 °C rotating incubator. Reverse transcriptase PCR Total RNA was extracted from LCM-collected CM, RPE and NE and from the whole eye and liver at E4 and E18, respectively. Total RNA was isolated using a NucleoSpin RNA II isolation Kit (Macherey-Nagel, Düren, Germany). Approximately 300 ng of total RNA from the whole eye and liver were used for complementary DNA synthesis using an ImProm-II Reverse Transcription System (Promega) and random-primer hexamers according to the manufacturer’s instructions. In case of CM, RPE and NE, the amplified SPIA (single primer isothermal amplification) cDNA was used as a template in the PCR reactions [48] . All PCR reactions were performed using PlatinumTaq DNA polymerase (Invitrogen) and the primers are listed in the Supplementary Table S1 . Amplification conditions included: denaturation at 95 °C for 1 min, annealing at 55 °C for 2 min and extension at 72 °C for 30 s. All the RT–PCR reactions were run using at least three independent biological samples. Peptide synthesis and antibody production The peptides and rabbit antibodies used in this study were produced using established methods as described [7] . Supplementary Table S2 contains the sequences of the peptides and antigens used to make antibodies ( Supplementary Fig. S3 ). Recombinant chicken C3a was cloned in pQE30 (Qiagen) and expressed according to the manufacturer's instructions. The recombinant C3a and the C-terminus C3a peptide (C3a-p) were designed on the basis of the sequence with accession number NP_990736. The Scr (control) peptide has the same amino-acid content as C3a-p but the sequence is scrambled. The C5a C-terminus peptide (C5a-p) was designed on the basis of the predicted C5 sequence with accession number XP_415405.2. The C3aR peptide comes from the sequence with accession number NP_001025940. It was designed to be in the extracellular part of the molecule (in extracellular loop 2), based on alignment with C3aR from other species using ClustalW 2.0. 12 and on predictions by the tools HHMTOP [28] , [49] and TMpred (EMBnet) regarding the topology of the transmembrane regions ( Supplementary Fig. S3 ). Western analysis The presence of C3 and fragments of C3 as well as C3aR were detected by standard western blotting procedures using a 10% gel under reducing conditions, followed by transfer to a PVDF membrane using a semi-dry or wet transfer system. After the membranes were blocked in 4% non-fat milk in 10 mM sodium phosphate, pH 7.4, with 150 mM NaCl and 0.05% Tween 20, they were incubated with 0.5 μg ml −1 of the corresponding primary antibody followed by an incubation in a 1:5,000 dilution (in blocking solution) of secondary anti-rabbit antibody conjugated to horseradish peroxidase (Bio Rad). Detection was performed using chemiluminescence (Immobilon Western detection reagents; Millipore). Densitometry measurements are provided in Supplementary Table S3 . The phosphorylation of STAT3 at serine 727 was detected by standard western blotting technique using a 10% SDS-PAGE gel followed by wet transfer to a PVDF membrane. Antibodies against pS727 STAT3 (1:1,000 dilution) and actin (1:1,000 dilution) were purchased from Cell Signaling Technology, Inc. (Danvers, MA) and Sigma-Aldrich (St Louis, MO) respectively. Secondary antibodies were purchased from Molecular Probes, Inc. (Eugene, OR). Detection was performed using chemiluminescence (Immobilon Western detection reagents; Millipore). Protein was collected using RIPA buffer plus protease inhibitors (Santa Cruz Biotechnologies, Santa Cruz, CA) from the CM 2 h PR and the appropriate treatments added. The CM was separated from the lens and cornea. At least five independent biological samples (CM of 25 pooled eyes equals one biological sample) were collected for each treatment. Densitometry was measured with ImageQuant, and the ratio of pS727 STAT3/actin was determined. Images of the western blots are provided in Supplementary Fig. S6 . Densitometry measurements are provided in Supplementary Table S3 . Laser-capture microdissection Embryos were collected at 2, 6 or 24 h post retinectomy and infiltrated at 4 °C with sucrose at 6.25%, 12.5% and 25% for 10, 20 or 30 min, respectively, equilibrated in 2:1 25% sucrose: OCT for 1 h and frozen in a mixture of dry ice and methylbutane. Cryosections (12 μm) were mounted onto metal-framed PEN membrane slides (Arcturus, Applied Biosystems), fixed in 70% ethanol at −20 °C, rinsed in DEPC-treated water, stained with hematoxylin for 10 s and dehydrated in 70% and 95% ethanol for 30 s and 100% ethanol for 2 min. LCM was carried out using a Veritas Laser-Capture Microdissection system and software (Molecular Devices) using Nikon × 20 affinity-corrected objectives with laser cutting (beam size of 2 mm, 7.5–8.0 mV) and laser capture (beam size of 5 mm, 70–100 mV). All sections (6 serial CM collections for each biological sample) were collected in CapSure HS LCM Caps (Molecular Devices) and RNA extraction was performed using a PicoPure RNA Isolation Kit (Arcturus, Applied Biosystems) including a treatment with DNase I (RNase-Free DNase Set, Qiagen). The quality and quantity of RNA were determined using an Agilent RNA 6000 pico LabChip (Agilent 2100 Bioanalyzer, Agilent Technologies). In general, samples showed a RNA integrity number (RIN)>8. Thereafter, 5 ng of total RNA were amplified using the Ovation Pico WTA System V2 (NuGEN, San Carlo, CA, USA). This linear and isothermal pre-amplification method started with randomly primed whole-transcriptome double-stranded cDNA synthesis followed by SPIA-based DNA pre-amplification to generate a final product of single-stranded cDNA product [48] . SPIA cDNA was purified using a QIAquick PCR Purification Kit (Qiagen) and quantified using a Nanodrop ND-100 spectrophotometer (Thermo Fisher Scientific). Reverse transcriptase quantitative PCR Reverse transcriptase quantitative PCR (RT–qPCR) was performed using a mixture (20 μl) containing 5 μl (4 ng) SPIA cDNA, 10 μl 2 × SYBR Green/Fluorescein qPCR Master Mix (SABiosciences, Qiagen) and a 500 nM final concentration of primers. Splice junction-specific primers were optimized following guidelines for RT–qPCR experiments, including the PCR amplification efficiency and melting curves [50] . All primers were designed using Primer 3 (v 4.0), available at http://primer3.wi.mit.edu/ . Primers sequences and Ensembl or GenBank IDs are provided in the Supplementary Table S4 . Amplifications reactions were performed (in triplicate) in an iCycler (Bio-Rad), and the cycling conditions included 10 min of polymerase activation at 95 °C and 35 cycles of 15 s at 95 °C and 1 min at 60 °C, followed by a dissociation run from 65 °C to 95 °C for melting curve analysis. All analyses were performed in triplicate with at least three independent biological samples. Average relative expression levels are provided in Supplementary Tables S5 and S6 . Surgical procedure Retinectomies were performed by removing the eggshell and embryonic membranes covering the eye of E4 embryos (HH stage 22–24). The eye was opened by cutting around the CM to produce a flap. The CM flap was pulled back and the retina removed. At this point, treatments were added to the vitreous chamber and the CM flap was closed. For C3a-p, C3a, C5a-p and Scr-treated eyes, 50 or 100 μg was injected into the vitreous chamber immediately following retinectomy. For FGF2-treated eyes, heparin beads containing FGF2 were prepared by incubating 20 heparin beads in 25 ng of FGF2 (R&D Systems, Minneapolis, MN) for 1 h at 4 °C and then added to the vitreous chamber. For IL-6-treated eyes, 25 ng of IL-6 was injected into the vitreous chamber immediately following retinectomy. C3a-p inhibition studies were performed by injecting a 6-μl aliquot of either 1 μM of PD173074 (Cell Signaling Technology, Inc., Danvers, MA), 1 μM of PD98059 (Cell Signaling Technology, Inc., Danvers, MA), 2 μM of Stattic (Tocris, Minneapolis, MN), 10 μM CHIR 99021 (Stemgent, San Diego, CA), 6 μg of C3aR-Ab or 30 ng of IL-6 Ab (AbD Serotec, Kidlington, UK) into the vitreous chamber post retinectomy 30 min before adding 50 μg of C3a-p (1 nM), along with another dose of either 1 μM of PD173074, 1 μM of PD98059, 2 μM of Stattic, 10 μm CHIR 99021, 3 μg of C3aR-Ab or 30 ng of IL-6 Ab, respectively. For FGF2 inhibition studies, a 6-μl aliquot containing 1 μM PD173074, 1 μM PD98059 or 6 μg of C3aR-Ab was injected into the vitreous chamber post retinectomy 30 min before adding 1.25 μg of FGF2, along with another dose of either 1 μM of PD173074, 1 μM of PD98059 or 3 μg of C3aR-Ab, respectively. Controls involved injecting an equal volume of DMSO or DPBS, or an equal amount of IgG. For BrdU proliferation studies, 10 μl of a 10 μg ml −1 BrdU solution was injected over the eye of the embryo 1 h before collection. Eyes used for histological analysis were fixed in Bouin’s fixative, embedded in paraffin wax, stained with hematoxylin and eosin (H&E) and photographed using an Olympus BX-51 microscope. Quantification of histological sections ImagePro Plus software was used to quantify the amount of regeneration in histological sections. For each eye, a section from the middle containing the lens and the highest amount of regeneration was chosen for quantification. Then, the free-hand tool of ImagePro Plus software was used to trace the regeneration from the CM, and the length of the tracing was calculated by the software. Quantification for histological data is provided in Supplementary Table S7 . Antibodies Antibodies against Pax-6 (1:10), Napa-73 (1:100), AP-2 (1:5), visinin (1:100), vimentin (1:100), were obtained from the Developmental Studies Hybridoma Bank developed under the auspices of the NICHD and maintained by The University of Iowa, Department of Biological Sciences, Iowa City, IA, USA. Antibody against anti-BrdU (1:100) was purchased from Abcam (Cambridge, MA), and anti-Brn3a (1:10) antibody was purchased from Chemicon International, Inc. (Temeucla, CA). Anti-Chx-10 (1:250) antibody was purchased from ExAlpha (Shirley, MA). All secondary antibodies were purchased from Molecular Probes, Inc. (Eugene, OR). Anti-C3 (1:100) and anti-C3aR (1:100) were generated as described above. Immunohistochemistry Tissues were fixed in 4% paraformaldehyde, cryoprotected in 30% sucrose, embedded in OCT freezing medium (Sakura Finetek, Torrance, CA), and sectioned at 12 μm. Sections were permeablized with 1% saponin (for antibodies against C3a, C3aR, Chx-10, Pax-6, Napa-73, Brn3a, visinin, vimentin and AP-2) or 2 N HCl (for anti-BrdU antibody), blocked in 10% normal goat serum, and incubated with primary antibody overnight at 4 °C. Tissues were incubated in secondary antibody and coverslipped with Vectashield (Vector Laboratories, Burlingame, CA). Confocal images (size 1,024 × 1,024) were collected sequentially on a Zeiss 710 Laser Scanning Confocal System (Germany) using a × 20/0.80 NA WD=0.55 objective lens or EC Plan-Neofluar × 40/0.75 M27 objective lens. Results were confirmed using three different biological samples. Quantification of immunohistochemistry results was done by counting the number of immunopositive cells from the anterior or posterior region of three different confocal images (1,024 × 1,024 taken at × 40) from three different eyes and the average number determined. Quantification data from immunohistochemistry is provided in Supplementary Table S8 . TUNEL TUNEL was performed using the in situ cell death detection kit TMR-red (Roche Applied Sciences, Indianapolis, IN). CM explant cultures and CHIR 99021 treatment E4 embryos were placed in 1 × Hank’s Balanced Salt Solution in DEPC water, the anterior portion of the eye was removed including the cornea and lens, and CM explants were collected and placed in a 24-well plate containing culture media (DMEM/F12, 5 mM HEPES, 0.11% NaHCO 3 , 0.6% glucose and penicillin 100 U ml −1 , streptomycin 100 μg ml −1 ) and incubated at 37 °C, 5% CO 2 . After collection, the explants ( n =4) were treated with 10 μM of CHIR 99021 (Stemgent, San Diego, CA) dissolved in DMSO:DPBS (50:50 v/v). As controls, untreated and DMSO:DPBS (50:50 v/v) treated CM explants were also included. Total RNA was extracted from the CM after a 24-h treatment using a RNA II isolation Kit (Macherey-Nagel, Düren, Germany) according to the manufacturer’s protocol. The cDNA synthesis was performed as described in the RT–PCR section using 200 ng of Total RNA previously analysed by the 6000 nano LabChip (Agilent 2100 Bioanalizer). Statistics For RT-qPCR studies, the comparative cycle at threshold (2 −ΔΔCt ) and an unpaired Student’s t -test analysis was used to determine relative changes in transcript levels compared with GAPDH mRNA levels using SigmaPlot 8.0 Software [51] , [52] , [53] . A two-tailed permutation test for comparing mean response was used to determine statistical significance for all histological analysis of regeneration and for the number of immunopositive and TUNEL-positive cells. The exact binomial test was used to determine a significant change in all western analysis. Error bars represent s.e.m. The alpha level was set at 0.05. How to cite this article: Haynes, T. et al . Complement anaphylatoxin C3a is a potent inducer of embryonic chick retina regeneration. Nat. Commun. 4:2312 doi: 10.1038/ncomms3312 (2013)